TREX exposes the RNA-binding domain of Nxf1 to enable mRNA export The metazoan TREX complex is recruited to mRNA during nuclear RNA processing and functions in exporting mRNA to the cytoplasm. Nxf1 is an mRNA export receptor, which binds processed mRNA and transports it through the nuclear pore complex. At present, the relationship between TREX and Nxf1 is not understood. Here we show that Nxf1 uses an intramolecular interaction to inhibit its own RNA-binding activity. When the TREX subunits Aly and Thoc5 make contact with Nxf1, Nxf1 is driven into an open conformation, exposing its RNA-binding domain, allowing RNA binding. Moreover, the combined knockdown of Aly and Thoc5 markedly reduces the amount of Nxf1 bound to mRNA in vivo and also causes a severe mRNA export block. Together, our data indicate that TREX provides a license for mRNA export by driving Nxf1 into a conformation capable of binding mRNA. The Nxf1 protein (also known as Tap in humans and Mex67p in yeast [1] , [2] , [3] , [4] , Fig. 1a ), functions as an export receptor for mRNA. Human Nxf1 (hereafter referred to as Nxf1) binds RNA through an N-terminal arginine-rich RNA-binding domain (RBD) and this activity is essential for mRNA export [5] , [6] . Multiple arginines within the Nxf1 RBD are required for interaction with RNA in vitro and with poly(A) + RNA in vivo , and thus may provide a charged platform for RNA interactions [6] . The Nxf1 RBD displays no obvious sequence specificity and binds a variety of RNA substrates [5] , [6] . Once bound to mRNA, Nxf1 escorts the messenger ribonucleoprotein (mRNP) to the nuclear pore, where Nxf1 interacts with nucleoporins via the NTF2-like (NTF2L) and ubiquitin-associated (UBA) domains [7] . Normally, mRNA is only exported to the cytoplasm upon completion of mRNA processing, though how the cell orchestrates the timely export of mRNA through the Nxf1 pathway is not clear. 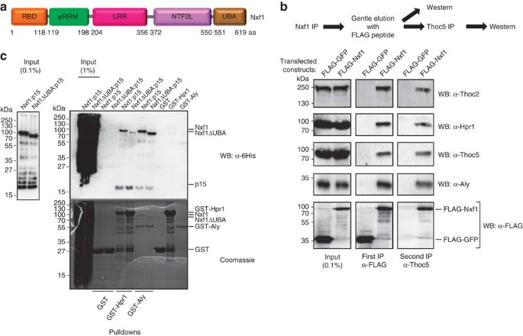Figure 1: Nxf1 and TREX assemble in a complexin vivo. (a) Schematic of Nxf1 showing its domains. ψRRM, pseudo RNA recognition motif; UBA, ubiquitin associated. (b) IP analysis of Nxf1. FLAG-Nxf1 was immunoprecipitated using FLAG antibody, eluted using FLAG peptide and then immunoprecipitated a second time using Thoc5 antibody. At each stage, samples were analysed by western blotting using the indicated antibodies. (c) The UBA domain of Nxf1 is required for interaction with Hpr1. GST-Hpr1 or GST-Aly pulldowns with the indicated Nxf1 constructs. Nxf1-GB1-6His or Nxf1ΔUBA-GB1-6His were co-expressed with p15-6His in BL21RPE. colistrain. Total extracts were prepared, cleared by centrifugation and used in pulldown experiments with GST-Hpr1 or GST-Aly in RB100 buffer in the presence of RNase A (10 μg ml−1). Pulldowns were analysed by SDS–PAGE followed by Coomassie staining or western blot using 6His antibody. aa, Amino acid. Figure 1: Nxf1 and TREX assemble in a complex in vivo . ( a ) Schematic of Nxf1 showing its domains. ψRRM, pseudo RNA recognition motif; UBA, ubiquitin associated. ( b ) IP analysis of Nxf1. FLAG-Nxf1 was immunoprecipitated using FLAG antibody, eluted using FLAG peptide and then immunoprecipitated a second time using Thoc5 antibody. At each stage, samples were analysed by western blotting using the indicated antibodies. ( c ) The UBA domain of Nxf1 is required for interaction with Hpr1. GST-Hpr1 or GST-Aly pulldowns with the indicated Nxf1 constructs. Nxf1-GB1-6His or Nxf1ΔUBA-GB1-6His were co-expressed with p15-6His in BL21RP E. coli strain. Total extracts were prepared, cleared by centrifugation and used in pulldown experiments with GST-Hpr1 or GST-Aly in RB100 buffer in the presence of RNase A (10 μg ml −1 ). Pulldowns were analysed by SDS–PAGE followed by Coomassie staining or western blot using 6His antibody. aa, Amino acid. Full size image The TREX complex [8] has an important but undefined molecular function in mRNA export. TREX comprises a core THO complex, which consists of Thoc2, Hpr1, Thoc5, Thoc6, Thoc7 and Tex1 in metazoans [9] , [10] and Tho2p, Hpr1p, Mft1p and Thp2p in yeast [11] . The human THO complex assembles in an ATP-dependent manner with the RNA helicase Uap56, Aly and Cip29 (ref. 12 ). The TREX complex is recruited to spliced mRNA [10] near the 5′ cap [13] . Furthermore, Yra1p, the yeast orthologue of Aly is delivered to the TREX complex during 3′-end processing by Pcf11p, and the Pcf11–Aly interaction is conserved in humans [14] . Two TREX components, Aly and Thoc5, bind directly to Nxf1. Aly associates with the N-terminal RBD and adjacent ψRRM of Nxf1 ( Fig. 1a ) [15] and this interaction is conserved in yeast [16] . Aly binds RNA via an arginine-rich peptide [17] that doubles as the binding site for Nxf1. When Nxf1 is recruited to an Aly:RNA complex, the RNA is handed over from Aly to Nxf1, and Aly enhances the RNA-binding activity of Nxf1 by an undefined mechanism [6] . The NTF2L domain of Nxf1 ( Fig. 1a ) binds Thoc5 in vitro , and Thoc5 and Aly bind simultaneously to Nxf1 in vitro , though the functional consequences of Thoc5 binding are not clear [18] . Finally, in yeast, Hpr1p associates with the C-terminal UBA domain of Mex67p, which is conserved in Nxf1. This interaction is enhanced by Hpr1 ubiquitinylation and drives recruitment of Mex67p to sites of transcription [19] . Nxf1 and TREX exist on the same mRNP [18] , though these interactions may be bridged by mRNA, and it is not clear whether Nxf1 associates via protein–protein interactions with assembled TREX in vivo. In yeast, loss of TREX components triggers a rapid mRNA export block [8] though RNAi of most metazoan TREX components results in a less striking mRNA export block [18] , [20] . The protein Uif, whose abundance increases significantly following Aly RNAi, compensates for Aly knockdown [20] . Consistent with these data, double knockdown of Aly and Uif potently blocks mRNA export, resulting in cell death in 6 days. Here we provide evidence that Nxf1 inhibits its own RNA-binding activity via an intramolecular interaction and that TREX components function to expose Nxf1's RBD, thereby allowing binding of the RNA to Nxf1. Thoc5 and Aly are essential for this process, and knockdown of these two proteins significantly reduces the amount of Nxf1 bound to mRNA in vivo . These results suggest that TREX is the major complex used to recruit Nxf1 to mRNA in human cells. TREX acts as a binding platform for Nxf1 To determine whether Nxf1 associates with an assembled TREX complex, we immunoprecipitated Nxf1 from a cell extract treated with RNase A to disrupt protein interactions bridged via RNA ( Supplementary Fig. S1 ). Following immunoprecipitation (IP), proteins were eluted under native conditions and identified by western blotting. This analysis revealed that multiple TREX components co-IP with Nxf1 ( Fig. 1b ). To determine whether these proteins were assembled in a single complex with Nxf1 or in multiple complexes, a secondary IP with Thoc5 antibody was carried out using the Nxf1 IP as starting material. Significantly, the secondary IP also contained Nxf1 and TREX components, indicating they can assemble into a single complex in vivo . We further established that Hpr1 binds Nxf1 ( Fig. 1c ) and this interaction is significantly reduced when the UBA domain is removed, indicating that the UBA domain has an important role in the interaction with Hpr1 as it does in yeast [19] . Thus, TREX components Aly, Thoc5 and Hpr1 make contact with Nxf1. Thoc5 and Aly disrupt an Nxf1 intramolecular interaction The Nxf1 domains are separated by flexible linkers [7] , [21] , [22] , [23] offering the possibility of conformational changes to Nxf1 on binding TREX. To examine this, we first carried out pulldown assays and found that GST-Nxf1:p15 interacts with full-length Nxf1 and the isolated RBD and NTF2L domains ( Fig. 2a , lanes 2–9). To investigate whether Nxf1:p15 might form an interdomain interaction between the RBD and NTF2L domains, we carried out a pulldown assay with the GST-NTF2L domain bound to p15 ( Fig. 2a , lanes 10–12). Full-length Nxf1 bound GST-NTF2L:p15 as did the RBD. This indicates that the NTF2L domain forms an interdomain interaction with the RBD. The leucine-rich repeat (LRR), ψRRM and UBA domains did not show any binding activity in these experiments. Therefore, we cannot exclude the possibility that these domains were non-functional or only partially functional. However, the UBA domain did bind a NUP214 fragment, indicating it retains some activity ( Supplementary Fig. S2 ). As a further control, we confirmed that the RBD used in these studies retained RNA crosslinking activity, moreover this activity is conserved within amino acids 1–112 of Drosophila melanogaster Nxf1 ( Fig. 2b ), which also contains an arginine-rich region ( Fig. 2c ). 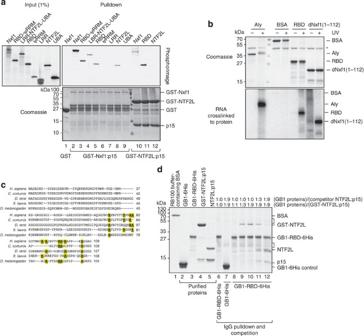Figure 2: The NTF2L domain of Nxf1 sequesters the RNA-binding domain. (a) GST pulldowns with the indicated GST fusions and domains of Nxf1 synthesized and35S-radiolabeledin vitroin reticulocyte lysate. (b) RNA-binding activity of the indicated constructs was analysed by ultraviolet light (UV)-crosslinking. dNxf1:D. melanogasterNxf1 protein. The asterisk designates the RNase inhibitor present in the reactions. (c) TheHomo sapiensN-terminal RBD sequence is aligned with the equivalent sequences from other metazoa. Within theH. sapienssequence, 10 arginines have been shown to be essential for the RNA-binding activityin vitro, poly(A)+RNA associationin vivoand mRNA export6. These are highlighted in yellow in the alignment as are equivalent residues in other Nxf1 sequences. In all metazoa, the sequences, which align with theH. sapiens35 amino acid arginine-rich sequence involved in RNA binding, show a strong bias towards arginine residues as follows:H. sapiens10/35 amino acids=29% arginine,Coturnix coturnix, 6/26 amino acids=23% arginine,D. rerio10/37 amino acids=27% arginine,Xenopus laevis,6/33 amino acids=18% arginine andD. melanogaster, 6/30=20% arginine. (d) Binding of the NTF2L domain to the RBD is direct. Binding of the NTF2L domain to the RBD was analysed by an immunoglobulin (IgG)-pulldown experiment performed in RB100 buffer in the presence of BSA (lane 1) and RNase A using purified GB1-6His or GB1-RBD-6His and GST-NTF2L:p15 (lanes 7–12). Unbound proteins were washed away and subsequently either buffer (lanes 8–10) or NTF2L:p15 competitor (lanes 7, 11 and 12) was added at the indicated molar ratios. The GB1 tag binds IgG beads. Purified proteins used in this assay are shown in lanes 2–5. Bound proteins were eluted and subsequently analysed by SDS–PAGE and Coomassie staining. Lane 6 shows IgG binding and elution of GB1-RBD-6His alone, performed in the same conditions as the pulldown assays. Additional bands, not present in the GB1-RBD-6His input sample, arising from the IgG beads are marked on the right hand side of the gel by brackets. Figure 2: The NTF2L domain of Nxf1 sequesters the RNA-binding domain. ( a ) GST pulldowns with the indicated GST fusions and domains of Nxf1 synthesized and 35 S-radiolabeled in vitro in reticulocyte lysate. ( b ) RNA-binding activity of the indicated constructs was analysed by ultraviolet light (UV)-crosslinking. dNxf1: D. melanogaster Nxf1 protein. The asterisk designates the RNase inhibitor present in the reactions. ( c ) The Homo sapiens N-terminal RBD sequence is aligned with the equivalent sequences from other metazoa. Within the H. sapiens sequence, 10 arginines have been shown to be essential for the RNA-binding activity in vitro , poly(A) + RNA association in vivo and mRNA export [6] . These are highlighted in yellow in the alignment as are equivalent residues in other Nxf1 sequences. In all metazoa, the sequences, which align with the H. sapiens 35 amino acid arginine-rich sequence involved in RNA binding, show a strong bias towards arginine residues as follows: H. sapiens 10/35 amino acids=29% arginine, Coturnix coturnix , 6/26 amino acids=23% arginine, D. rerio 10/37 amino acids=27% arginine, Xenopus laevis, 6/33 amino acids=18% arginine and D. melanogaster , 6/30=20% arginine. ( d ) Binding of the NTF2L domain to the RBD is direct. Binding of the NTF2L domain to the RBD was analysed by an immunoglobulin (IgG)-pulldown experiment performed in RB100 buffer in the presence of BSA (lane 1) and RNase A using purified GB1-6His or GB1-RBD-6His and GST-NTF2L:p15 (lanes 7–12). Unbound proteins were washed away and subsequently either buffer (lanes 8–10) or NTF2L:p15 competitor (lanes 7, 11 and 12) was added at the indicated molar ratios. The GB1 tag binds IgG beads. Purified proteins used in this assay are shown in lanes 2–5. Bound proteins were eluted and subsequently analysed by SDS–PAGE and Coomassie staining. Lane 6 shows IgG binding and elution of GB1-RBD-6His alone, performed in the same conditions as the pulldown assays. Additional bands, not present in the GB1-RBD-6His input sample, arising from the IgG beads are marked on the right hand side of the gel by brackets. Full size image We confirmed that the RBD:NTF2L:p15 interaction was direct and reversible using pulldown assays with domains purified from Escherichia coli ( Fig. 2d ). Binding of GST-NTF2L:p15 to GB1-RBD-6His was direct ( Fig. 2d , lanes 8–10), and specific as it was reversed by additions of the purified competitor NTF2L:p15 ( Fig. 2d lanes 11 and 12). In Fig. 2d lane 7, a GB1-6His control construct was used in a pulldown with GST-NTF2L:p15 at a molar ratio 1:9 (GB1-6His/GST-NTF2L:p15), washed and subsequently the competitor NTF2L:p15 was added at a molar ratio 1:9 (GB1-6His/NTF2L:p15). No GST-NTF2L:p15 or NTF2L:p15 are seen following pulldown indicating that these proteins do not bind nonspecifically to either GB1-6His or the beads. As the purified GB1-RBD-6His fragment of Nxf1 used in these assays has some visible minor truncations, we cannot exclude the possibility that these also contribute to the binding of GST-NTF2L:p15 ( Fig. 2d , lanes 8–10) or NTF2L:p15 ( Fig. 2d , lanes 11 and 12). To define the surface of the NTF2L domain bound by the RBD, we examined the interaction using a mutant NTF2L domain (456KHTR459 changed to 456AAAA459), which no longer binds Thoc5 [18] . These mutations lie on the opposite face of the NTF2L domain to that which binds p15 ( Fig. 3a,b ) and do not alter the interaction with p15 ( Fig. 3c and ref. 18 ). Surprisingly, we found that these NTF2L domain mutations enhance the interaction with the RBD ( Fig. 3c ). To define further residues required for the RBD:NTF2L interaction, we generated additional mutations in the NTF2L domain. These mutations did not prevent p15 or a NUP214 fragment from binding the NTF2L domain, suggesting the overall fold of the domain is not perturbed ( Supplementary Fig. S2 ). The R453D and the double-mutant K456D-R459D significantly reduced the GST-RBD:NTF2L interaction ( Fig. 3d ). These residues cluster on the same surface that binds Thoc5 and opposite the face that binds p15 ( Fig. 3b ). Consistent with this, p15 is not required for the interaction between GST-RBD and the NTF2L domain ( Fig. 3d , lane 2). The ability of the NTF2L R453D and K456D-R459D mutations to reduce the NTF2L:RBD association, together with the ability of the 456AAAA459 mutations to enhance binding, indicate this surface of the NTF2L domain is responsible for specific binding to the RBD. 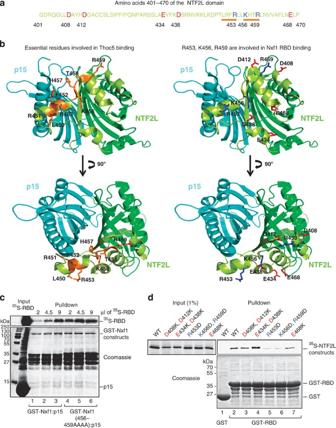Figure 3: Identification of the NTF2L:RBD-binding interface. (a) Sequence of the region of the NTF2L domain targeted by the mutagenesis. Targeted residues are highlighted as red for acidic and blue for basic. Orange bars indicate the most crucial residues involved in Thoc5 binding18that also enhance Nxf1 interdomain interaction when mutated to alanines (in case of 456–459). (b) Positions of the above mentioned residues on NTF2L:p15 structure (1JKG) using the same colours as in (a). p15 is presented in cyan colour, the NTF2L domain is presented in dark green colour and targeted region within the NTF2L domain is presented in light green colour. (c) Nxf1 (456–459AAAA) mutant binds Nxf1 RBD more efficiently than wild-type Nxf1. GST pulldowns with the indicated fusions and increasing amounts of35S-RBD. (d) GST-pulldown experiment using GST-RBD and the indicatedin vitrotranslated mutants of the NTF2L domain of Nxf1. Figure 3: Identification of the NTF2L:RBD-binding interface. ( a ) Sequence of the region of the NTF2L domain targeted by the mutagenesis. Targeted residues are highlighted as red for acidic and blue for basic. Orange bars indicate the most crucial residues involved in Thoc5 binding [18] that also enhance Nxf1 interdomain interaction when mutated to alanines (in case of 456–459). ( b ) Positions of the above mentioned residues on NTF2L:p15 structure (1JKG) using the same colours as in ( a ). p15 is presented in cyan colour, the NTF2L domain is presented in dark green colour and targeted region within the NTF2L domain is presented in light green colour. ( c ) Nxf1 (456–459AAAA) mutant binds Nxf1 RBD more efficiently than wild-type Nxf1. GST pulldowns with the indicated fusions and increasing amounts of 35 S-RBD. ( d ) GST-pulldown experiment using GST-RBD and the indicated in vitro translated mutants of the NTF2L domain of Nxf1. Full size image Normally, it would be expected that intramolecular interactions between the NTF2L domain and the RBD would prevail over intermolecular interactions, yet the pulldown assay with Nxf1 and fragments does not distinguish these possibilities and only confirm that an interdomain interaction can occur. Thus, we examined Nxf1:p15 migration by gel filtration ( Supplementary Fig. S3 ) and found that the majority of Nxf1:p15 behaves as a heterodimer (one molecule of Nxf1 complexed with one molecule of p15). Therefore, the intramolecular interaction predominates, though this experiment does not establish the proportion of the NTF2L and RBD domains bound to each other in free Nxf1. It was previously suggested that Nxf1 forms oligomers [24] , based on gel filtration of Nxf1 generated in reticulocyte lysate, though the high apparent molecular weight observed for Nxf1 in these earlier experiments could be explained by its association with other protein complexes in reticulocyte lysate. Thoc5 and Aly bind the two Nxf1 domains implicated in the Nxf1 interdomain interaction. Therefore, we investigated whether they might influence this interaction. GST-Nxf1:p15 pulls down 35 S-Nxf1 ( Fig. 4 ), and the addition of Aly or Thoc5 alone does not prevent this interaction. However, their combined presence does. Moreover, in the presence of Aly, more Thoc5 associates with Nxf1, as reported previously [18] . Together, these data suggest that Thoc5 and Aly binding can disrupt the closed conformation of Nxf1. 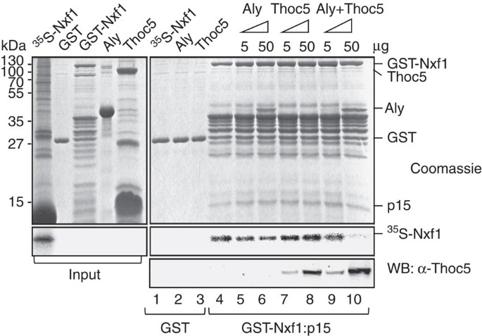Figure 4: Both Aly and Thoc5 are required to disrupt Nxf1–Nxf1 interactions. Pulldown assays with GST-Nxf1:p15 and35S-radiolabeled Nxf1 in the presence of the indicated TREX components. The lower panel is a western blot to detect the binding of Thoc5. All of these experiments were carried out in the presence of RNase A. Figure 4: Both Aly and Thoc5 are required to disrupt Nxf1–Nxf1 interactions. Pulldown assays with GST-Nxf1:p15 and 35 S-radiolabeled Nxf1 in the presence of the indicated TREX components. The lower panel is a western blot to detect the binding of Thoc5. All of these experiments were carried out in the presence of RNase A. Full size image Nxf1 RNA binding is regulated by an intramolecular interaction As the Nxf1 interdomain interaction involves its RBD, we investigated what impact this interaction has on Nxf1 RNA-binding activity. Using ultraviolet crosslinking with purified proteins and 5′-radiolabelled 15-mer RNA, we found that amino acids 1–372 of Nxf1, including the RBD, but lacking the NTF2L domain, crosslinks with RNA more efficiently than full-length Nxf1 ( Fig. 5a ). Moreover, when an Nxf1 fragment containing the RBD is affinity purified using the NTF2L domain fused to GST, and is therefore fully saturated with NTF2L domain, it fails to crosslink with RNA ( Fig. 5b , lanes 6 and 7) whereas the free Nxf1 fragment containing the RBD binds RNA efficiently ( Fig. 5b , lanes 1–5). In these experiments, we used a GST pulldown as a control ( Fig. 5b , lanes 10 and 11) to confirm that the RBD is specifically binding GST-NTF2L rather than nonspecifically precipitating with glutathione sepharose. Together, these data indicate that the RBD:NTF2L interdomain interaction inhibits Nxf1's RNA-binding activity. However, given that free Nxf1 is able to crosslink with RNA weakly, at steady state a proportion of Nxf1 is in an open conformation. Significantly, the NTF2L domain mutations, Nxf1 (456–459AAAA), which enhance the Nxf1 interdomain interaction, also reduce the ability of full-length Nxf1 to crosslink with RNA in vitro ( Fig. 5c ). As the in vitro RNA-binding studies were carried out with an RNA oligonucleotide ( Fig. 5a–c ), we cannot exclude the possibility that the interaction of Nxf1 with mRNA in vivo might differ in its behaviour. However, Nxf1 (456–459 AAAA) also reduced the association of Nxf1 with the mRNP in vivo ( Fig. 5d ). Similarly, a mutant form of Nxf1, which harbours 10 arginine to alanine mutations in the RBD (10RA) and fails to bind the RNA used in these studies [6] , also fails to associate with poly(A) + RNA in vivo ( Fig. 5d and ref. 6 ). Therefore, the Nxf1 (456–459 AAAA) mutations impaired Nxf1 RNA-binding activity both in vitro and in vivo . To further examine the effects of the Nxf1 (456–459AAAA) mutations on mRNA export, we used an RNAi complementation assay [6] . A wild-type Nxf1 cDNA resistant to RNAi efficiently complements an Nxf1 knockdown and restores normal mRNA export. However, the RBD mutant Nxf1(10RA) [6] or the Nxf1 (456–459AAAA) mutations, both of which fail to bind RNA efficiently in vitro and in vivo , fail to complement Nxf1 RNAi, resulting in a robust nuclear accumulation of poly(A) + RNA in these cells ( Fig. 5e ). Together, these data indicate that Nxf1 RNA-binding activity is regulated by its interdomain interaction. 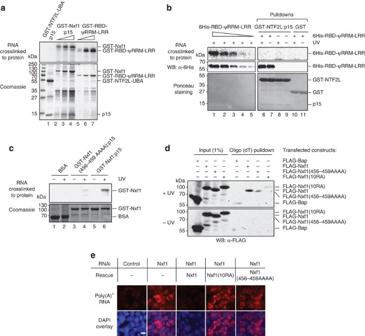Figure 5: The Nxf1 intramolecular interaction regulates its RNA-binding activity. (a) RNA crosslinking activity for GST-TAP:p15 and GST-RBD-ψRRM-LRR. The three different Nxf1 construct protein concentrations used (from left to right) were 88, 265 and 530 nM and the RNA concentration was 6.5 μM. (b) The Nxf1 RBD fails to bind RNA when complexed with the NTF2L domain. The 6His-RBD-ψRRM-LRR protein efficiently crosslinks with RNA (top panel lanes 1–5, using 200, 100, 50, 20 and 10 ng of protein). RNA binding was detected by phosphoimaging. 6His-RBD-ψRRM-LRR was detected by western blot (middle panel) and the GST constructs were detected by Ponceau staining (bottom panel). (c) RNA crosslinking activity for GST-Nxf1 (456–459AAAA):p15 and GST-Nxf1:p15. RNA binding was detected by phosphoimaging. (d) mRNP capture assay with indicated Nxf1 constructs. Bap is bacterial alkaline phosphatase control. Nxf1(10RA) is a mutant form of Nxf1, which is unable to bind RNA efficiently6. (e) RNA export assay in 293T cells. Cells were transfected with the Nxf1 RNAi vector together with the indicated rescue Nxf1 expression vectors, resistant to RNAi. Cells were analysed by fluorescentin situhybridisation (FISH) with Cy3-oligo(dT) (top panel) and images overlayed with 4',6-diamidino-2-phenylindole (DAPI) staining of the same cells (bottom panel). All pictures were taken at the same exposure level. The white horizontal bar represents 10 μm. Figure 5: The Nxf1 intramolecular interaction regulates its RNA-binding activity. ( a ) RNA crosslinking activity for GST-TAP:p15 and GST-RBD-ψRRM-LRR. The three different Nxf1 construct protein concentrations used (from left to right) were 88, 265 and 530 nM and the RNA concentration was 6.5 μM. ( b ) The Nxf1 RBD fails to bind RNA when complexed with the NTF2L domain. The 6His-RBD-ψRRM-LRR protein efficiently crosslinks with RNA (top panel lanes 1–5, using 200, 100, 50, 20 and 10 ng of protein). RNA binding was detected by phosphoimaging. 6His-RBD-ψRRM-LRR was detected by western blot (middle panel) and the GST constructs were detected by Ponceau staining (bottom panel). ( c ) RNA crosslinking activity for GST-Nxf1 (456–459AAAA):p15 and GST-Nxf1:p15. RNA binding was detected by phosphoimaging. ( d ) mRNP capture assay with indicated Nxf1 constructs. Bap is bacterial alkaline phosphatase control. Nxf1(10RA) is a mutant form of Nxf1, which is unable to bind RNA efficiently [6] . ( e ) RNA export assay in 293T cells. Cells were transfected with the Nxf1 RNAi vector together with the indicated rescue Nxf1 expression vectors, resistant to RNAi. Cells were analysed by fluorescent in situ hybridisation (FISH) with Cy3-oligo(dT) (top panel) and images overlayed with 4',6-diamidino-2-phenylindole (DAPI) staining of the same cells (bottom panel). All pictures were taken at the same exposure level. The white horizontal bar represents 10 μm. Full size image Thoc5 and Aly stimulate Nxf1 RNA binding To establish whether Thoc5 and Aly regulate Nxf1 RNA binding, we carried out ultraviolet crosslinking assays. Both Thoc5 and Aly crosslink with RNA in vitro , although Thoc5 crosslinks less efficiently than Aly ( Fig. 6a , lanes 1–6). Nxf1 also crosslinks weakly with RNA. However, in the presence of Thoc5 alone, the crosslink on Nxf1 is lost ( Fig. 6a , lane 10). In the absence of Aly, Nxf1 remains a poor RNA crosslinker [6] and it is likely that the radiolabelled RNA, sequestered by the unbound Thoc5, was washed away before elution of the protein:RNA complex and ultraviolet crosslinking (Methods). Nevertheless, this result shows that Thoc5 alone does not enhance the RNA-binding activity of Nxf1. In complex with Nxf1:p15, Aly stimulates Nxf1 RNA binding ( Fig. 6a , lane 12), as reported previously [6] . The combination of Aly and Thoc5 further stimulates Nxf1's binding to RNA ( Fig. 6a , lane 14), indicating both proteins are required for optimal Nxf1:RNA interactions. To investigate the contribution of Aly and Thoc5 to Nxf1:mRNA interactions in vivo , we used an mRNP capture assay. Stable knockdown of either Aly or Thoc5 ( Supplementary Fig. S4 ) did not prevent the Nxf1:mRNA interaction ( Fig. 6b ). However, double knockdown of Aly and Thoc5 led to a marked reduction in the amount of Nxf1 bound to mRNA in vivo ( Fig. 6b ), consistent with the ability of these proteins to disrupt the Nxf1 intramolecular interaction and expose its RBD. In contrast, the interaction of Uap56 with mRNA was not affected by Thoc5 and Aly RNAi ( Fig. 6b ), consistent with Uap56 functioning upstream of these TREX components in the mRNA export pathway [20] , [25] . We further investigated the effects of Aly and Thoc5 knockdown on mRNA export and found that, as reported previously [18] , [20] , single knockdown of Aly or Thoc5 had a modest impact on mRNA export ( Fig. 6c ), consistent with Nxf1's ability to bind mRNA under these conditions ( Fig. 6b ). In contrast, the Aly+Thoc5 combined knockdown caused a rapid and extreme mRNA export block ( Fig. 6c ), which led to cell death after 5 days. As Thoc5 RNAi has a minimal impact on bulk mRNA export ( Fig. 6c and ref. 18 ), these results rule out the possibility that the Nxf1 (456–459AAAA) construct fails to complement Nxf1 RNAi ( Fig. 5e ) because it cannot bind Thoc5. 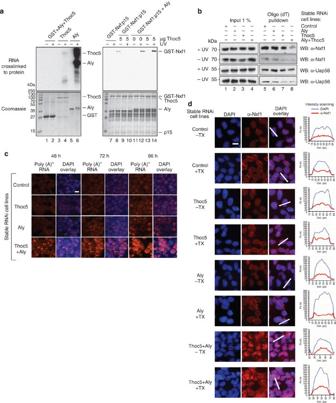Figure 6: Thoc5 and Aly trigger Nxf1 opening allowing RNA binding and efficient mRNA export. (a) Nxf1 remodelling assay. The indicated protein complexes were formed and UV crosslinked with a 5′-radiolabeled RNA. The top panels are phosphoimages and the bottom panels are their corresponding gels coomassie stained. (b) mRNP capture assay shows that Aly and Thoc5 knockdown prevents efficient recruitment of Nxf1 to mRNA. miRNA expression was induced for 48 h before analysis. (c) Oligo(dT) FISH on stable 293 cell lines expressing miRNAs targeting the indicated genes. The time points refer to the time following induction of the miRNA expression. Cells were treated with actinomycin D for 2 h before FISH to reduce nascent RNA signals. All pictures are taken at the same exposure level. (d) Nuclear envelope association of Nxf1 is impairedin vivowhen both TREX components Aly and Thoc5 are depleted by RNAi. After 72 h of induction of miRNAs expression, the indicated 293 stable RNAi cell lines were subjected to TX extraction before fixation when indicated (+TX) and the localisation of Nxf1 was analysed by immunostaining α-Nxf1 and fluorescence intensity scanning (white bars and corresponding graphs). Theyaxis of the graphs represents the pixel intensity (Px Int.) and thexaxis the distance in pixels (Dist. (px)). The white horizontal bars in (c) and (d) represent 10 μm. Figure 6: Thoc5 and Aly trigger Nxf1 opening allowing RNA binding and efficient mRNA export. ( a ) Nxf1 remodelling assay. The indicated protein complexes were formed and UV crosslinked with a 5′-radiolabeled RNA. The top panels are phosphoimages and the bottom panels are their corresponding gels coomassie stained. ( b ) mRNP capture assay shows that Aly and Thoc5 knockdown prevents efficient recruitment of Nxf1 to mRNA. miRNA expression was induced for 48 h before analysis. ( c ) Oligo(dT) FISH on stable 293 cell lines expressing miRNAs targeting the indicated genes. The time points refer to the time following induction of the miRNA expression. Cells were treated with actinomycin D for 2 h before FISH to reduce nascent RNA signals. All pictures are taken at the same exposure level. ( d ) Nuclear envelope association of Nxf1 is impaired in vivo when both TREX components Aly and Thoc5 are depleted by RNAi. After 72 h of induction of miRNAs expression, the indicated 293 stable RNAi cell lines were subjected to TX extraction before fixation when indicated (+TX) and the localisation of Nxf1 was analysed by immunostaining α-Nxf1 and fluorescence intensity scanning (white bars and corresponding graphs). The y axis of the graphs represents the pixel intensity (Px Int.) and the x axis the distance in pixels (Dist. (px)). The white horizontal bars in ( c ) and ( d ) represent 10 μm. Full size image During mRNA export, Nxf1 associates with the FG repeats of nucleoporins at the nuclear pore and this can be detected by immunofluorescence in cells treated with Triton X-100 (TX), which allows release of the intranuclear Nxf1 [26] . As TREX components are required for the stable association of Nxf1 with the mRNP, we investigated whether they might also be required for the subsequent association of Nxf1 with the nuclear pore. In the absence of TX, Nxf1 shows a diffuse nuclear staining following a control RNAi treatment ( Fig. 6d ; Supplementary Fig. S5 ), whereas when cells are treated with TX, the diffuse intranuclear staining is reduced and the nuclear rim staining becomes prominent. This is also apparent when the fluorescence intensity across the nucleus is monitored, with clear peaks of Nxf1 staining at the nuclear rim ( Fig. 6d , graphs on the right hand side). Following either Thoc5 or Aly RNAi, the nuclear rim staining for Nxf1 is still visible. In contrast, combined RNAi of Aly+Thoc5 markedly reduced the nuclear rim association of Nxf1 and peaks of nuclear rim staining are not visible ( Fig. 6d , graph right hand side and Supplementary Fig. S5 ). Interestingly, the intranuclear staining for Nxf1 in the presence or absence of TX was also increased following Aly+Thoc5 RNAi. To confirm that TX efficiently released soluble proteins from the 293 cell nucleus, we monitored the green fluorescent protein signal produced by these stable RNAi cell lines and found consistently that TX treatment released GFP from these cells ( Supplementary Fig. S6 ). These data indicate that Aly and Thoc5 are required for the Nxf1 nuclear rim association and in their absence Nxf1 appears trapped in a TX release-resistant state. To further assess a requirement of TREX in allowing the recruitment of Nxf1 to the nuclear pores, we performed the TX release assay on cells stably knocked down for both Aly and the largest THO-TREX subunit Thoc2. The combination of Aly and Thoc2 RNAi reduced the nuclear rim staining for Nxf1 ( Fig. 7a ). Moreover, whereas Aly RNAi led to a modest mRNA export block, the combined RNAi of Aly and Thoc2 led to a potent mRNA export block, as severe as that seen following Nxf1 RNAi ( Fig. 7b ). Following Nxf1 RNAi, there is a concomitant increase in the levels of Thoc2 in cells ( Fig. 7c ). Such compensatory increases in mRNA export factors following RNAi of other export factors have been reported previously [2] , [20] and underscore the important functional relationship between TREX and Nxf1. 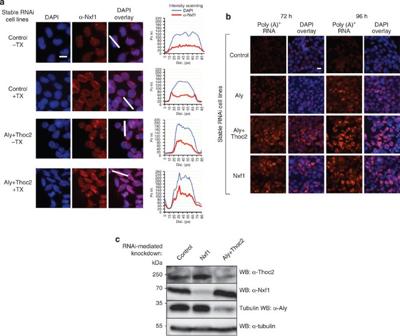Figure 7: Thoc2 has a role in Nxf1 localisation and mRNA export. (a) Nuclear envelope association of Nxf1 is impairedin vivowhen both TREX components Aly and Thoc2 are depleted by RNAi. Localisation of Nxf1 was analysed by immunostaining of control or (Aly+Thoc2) knockdown cell lines after 96 h of induction of miRNA expression using Nxf1 antibody. Where indicated (+TX), cells were treated with 0.5% TX before fixing. Theyaxis of the graphs represents the pixel intensity (Px Int.) and thexaxis the distance in pixels (Dist. (px)). (b) A strong block of bulk poly(A)+RNA export is observed in Nxf1 RNAi and (Aly+Thoc2) RNAi cell lines. Oligo (dT) fluorescentin situhybridisation (FISH) on stable 293 cell lines expressing miRNAs targeting the indicated genes. The time points refer to the time following induction of miRNAs expression. Cells were treated with actinomycin D for 2 h before FISH to reduce nascent RNA signals. All pictures are taken at the same exposure level. The white horizontal bars in (a) and (b) represent 10 μm. (c) Western blot analysis of the indicated cell lines. The expression of the miRNAs is under the control of a tetracycline inducible promoter. Extracts were prepared 96 h post-induction of miRNA expression and analysed using the indicated antibodies. Figure 7: Thoc2 has a role in Nxf1 localisation and mRNA export. ( a ) Nuclear envelope association of Nxf1 is impaired in vivo when both TREX components Aly and Thoc2 are depleted by RNAi. Localisation of Nxf1 was analysed by immunostaining of control or (Aly + Thoc2) knockdown cell lines after 96 h of induction of miRNA expression using Nxf1 antibody. Where indicated (+TX), cells were treated with 0.5% TX before fixing. The y axis of the graphs represents the pixel intensity (Px Int.) and the x axis the distance in pixels (Dist. (px)). ( b ) A strong block of bulk poly(A) + RNA export is observed in Nxf1 RNAi and (Aly+Thoc2) RNAi cell lines. Oligo (dT) fluorescent in situ hybridisation (FISH) on stable 293 cell lines expressing miRNAs targeting the indicated genes. The time points refer to the time following induction of miRNAs expression. Cells were treated with actinomycin D for 2 h before FISH to reduce nascent RNA signals. All pictures are taken at the same exposure level. The white horizontal bars in ( a ) and ( b ) represent 10 μm. ( c ) Western blot analysis of the indicated cell lines. The expression of the miRNAs is under the control of a tetracycline inducible promoter. Extracts were prepared 96 h post-induction of miRNA expression and analysed using the indicated antibodies. Full size image Our data lead to a model in which Nxf1 sequesters its N-terminal RBD, through an intramolecular interaction with its NTF2L domain. In this model ( Fig. 8 ), TREX binds to Nxf1, driving it into an open conformation, allowing it to stably bind mRNA and enable its export. Earlier studies have shown that RNAi of THO subunits leads to inhibition of mRNA export for a limited number of transcripts, including heatshock mRNAs [9] , [18] . In fact, depletion of Thoc5 in mouse cells only leads to a significant mRNA export block for ~2.9% of mRNAs [27] . Similarly, loss of Aly does not cause a strong mRNA export block [18] , [20] . We also find that loss of Thoc5 or Aly alone does not prevent the association of Nxf1 with mRNA in vivo ( Fig. 6 ), yet Nxf1 clearly binds an assembled TREX complex in vivo containing Aly and THO components ( Fig. 1 ). The failure to detect a strong export block in the absence of Aly may be due to Uif, which fulfils a similar role to Aly and is significantly upregulated in the cell in response to Aly RNAi [20] . Likewise, the ability of the cell to maintain recruitment of Nxf1 to mRNA in the absence of Thoc5 alone may be due to functional substitution by two other mRNA export factors that bind the Nxf1 NTF2L domain, Rbm15 and Rbm15B [28] . Despite redundant backup pathways to partially rescue mRNA export in the absence of single TREX components, disabling the TREX complex through RNAi of both Thoc5 and Aly largely prevents the binding of Nxf1 to mRNAs, leading to a concomitant rapid and lethal mRNA export block. Similarly knockdown of another THO complex component Thoc2 in combination with Aly RNAi leads to an mRNA export block. Together these data demonstrate an important role for the conserved THO–TREX complex in human mRNA export, although the precise repertoire of mRNAs that use the Nxf1 pathway in human cells still remains to be determined. 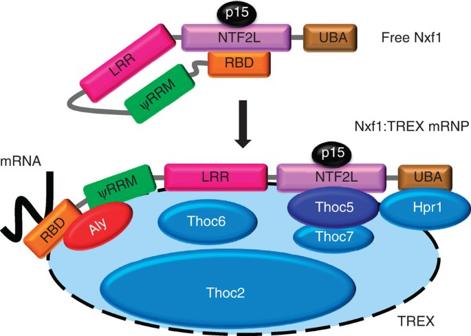Figure 8: A model for the conformational change in Nxf1 induced by TREX during mRNA export. Free Nxf1:p15 sequesters its N-terminal RBD. During mRNA export, assembled TREX binds Nxf1:p15. This allows the two subunits Aly and Thoc5 to remodel Nxf1 and expose its RBD, allowing direct interaction between Nxf1 and mRNA during export. For clarity not all TREX subunits are illustrated in the figure. Figure 8: A model for the conformational change in Nxf1 induced by TREX during mRNA export. Free Nxf1:p15 sequesters its N-terminal RBD. During mRNA export, assembled TREX binds Nxf1:p15. This allows the two subunits Aly and Thoc5 to remodel Nxf1 and expose its RBD, allowing direct interaction between Nxf1 and mRNA during export. For clarity not all TREX subunits are illustrated in the figure. Full size image The D. melanogaster orthologue of Nxf1 also harbours an N-terminal arginine-rich region that has RNA-binding activity ( Fig. 2b,c ) together with a conserved NTF2L domain [29] . Therefore, the regulation of Nxf1 RNA-binding activity may be conserved across metazoa. Whether the yeast counterpart of Nxf1, Mex67p, utilises a similar mechanism to bind mRNA and how this is controlled remain unclear as the N-terminal 100 amino acids of Mex67p does not show RNA-binding activity [21] . Furthermore, the Mex67p NTF2L domain and the p15 orthologue, Mtr2p, have extended positively charged loop sequences that interact with rRNA in vitro and allow Mex67p to participate in the nuclear export of the 60S ribosomal subunit [30] . These extended loop sequences are absent in Nxf1 and p15. Furthermore, yeast does not have a clear orthologue of THOC5. Therefore, these differences together with the lack of an apparent N-terminal RBD may partly explain the ability of Nxf1:p15 to only partially complement a Mex67:Mtr2 knockout [31] . There is a clear overlap between the RBD- and Thoc5-binding sites on the NTF2L domain of Nxf1 ( Fig. 3 ), yet only the combination of Thoc5 and Aly can unlock Nxf1 ( Fig. 4 ). Consistent with this observation, the weak binding of Thoc5 to Nxf1 in vitro is stimulated by Aly ( Fig. 4 and ref. 18 ). This suggests a two-stage mechanism for regulation of Nxf1 RNA binding whereby Aly partially destabilises the RBD interaction with the NTF2L domain, and this in turn facilitates Thoc5 binding and full displacement of the RBD from the NTF2L domain. As a consequence, maximal stimulation of Nxf1's RNA-binding activity is achieved. It is striking that the RBD:NTF2L domain interaction involves a cluster of NTF2L domain positively charged residues (R453, K456 and R459; Fig. 3 ), because Aly and SR proteins use a cluster of arginines to bind Nxf1 [6] , [32] , [33] . Such arginine-rich peptides from Aly or SR proteins may compete with R453, K456 and R459 from the NTF2L domain for interaction with the Nxf1 RBD, thus triggering its partial displacement from the NTF2L domain. Although the Nxf1 RBD has no predicted secondary structure, a recent report suggests that this domain self-associates [24] . Therefore, Aly may also cause local rearrangement of the RBD, although we have not observed disruption of the RBD self-association in the presence of Aly. Instead, the folding of the RBD into a tertiary structure may be a prerequisite for its interaction with the NTF2L domain and subsequent interaction with mRNA. Following combined knockdown of Aly and Thoc5, Nxf1 is no longer stably recruited to the mRNP. Furthermore, its nuclear rim association is reduced and a concomitant mRNA export block is observed. This implies that Nxf1 must be recruited to the mRNP to allow its subsequent docking at the nuclear pore and mRNA export. This may be because, upon recruitment to the mRNP, Nxf1 associates with proteins such as GANP, which promote its nuclear pore association [34] . When Nxf1 recruitment to the mRNP is disrupted, it accumulates in the nucleus in a TX insoluble fraction. We speculate that in this situation, Nxf1 becomes trapped with chromatin following its recruitment to transcription complexes via Hpr1 or other proteins and fails to be transferred to the mRNP via an assembled TREX complex. The constitutive transport element (CTE) of simple retroviruses binds Nxf1 with high affinity [35] and Nxf1 binds its own pre-mRNA, via a CTE-like structure within intron 10 [36] . In each case, the interaction involves the ψRRM and LRR domains [21] , [22] , [37] , [38] , which sit directly between the RBD and NTF2L domains. Therefore, it is conceivable that in order to bind Nxf1, the CTE has to disrupt the RBD:NTF2L interaction to gain access to the CTE-binding site. Intriguingly, 9G8, which is capable of remodelling Nxf1 and allowing it to bind mRNA more efficiently [6] , stimulates CTE activity in a translation assay [39] . Therefore, 9G8 may stimulate opening of Nxf1, facilitating CTE:Nxf1 interactions. In the structure of a fragment of Nxf1 bound to the CTE [38] , the concave surface of the LRR and the alpha helical surface of the ψRRM are exposed and do not make contact with the CTE. This leaves them available for interaction with proteins such as 9G8, which is known to bind the RBD-ψRRM fragment of Nxf1 [15] . Furthermore, there is a pronounced kink between the ψRRM and LRR domains of Nxf1 once bound to the CTE [38] , yet a significant proportion of the CTE is left solvent exposed. The authors speculated that the NTF2L and UBA domains and p15 may also contribute to the interaction with the CTE, by encapsulating it, as may the N-terminal RBD. Such a CTE encapsulating conformation for Nxf1 may bring the RBD and NTF2L domains into close proximity, similar to the closed conformation we propose here for free Nxf1. Alternatively, the model of two Nxf1 molecules bound to a full-length CTE [38] presents the Nxf1 molecules bound in a head to tail conformation on the CTE, which would potentially juxtapose the NTF2L and RBD domains from separate Nxf1 molecules, facilitating intermolecular NTF2L:RBD interactions and these may assist in establishing Nxf1:CTE interactions. Such a mode of Nxf1 binding the CTE would clearly diverge from the mechanism used by Nxf1 to bind cellular mRNA, yet suggests that the CTE might exploit the natural propensity of the Nxf1 RBD and NTF2L domains to interact for efficient binding. If Nxf1 is directly tethered to an unspliced pre-mRNA via an MS2 coat protein and operator, the pre-mRNA is exported to the cytoplasm without undergoing splicing [32] . Therefore, it is vital for the cell to regulate Nxf1's RNA-binding activity so that it only binds and exports processed mRNA. Our data indicate that Thoc5 and Aly regulate Nxf1 RNA-binding activity, providing a molecular timer, which ensures that Nxf1 is only loaded onto mRNA once these two proteins have assembled within TREX. TREX assembly is coupled with splicing [10] , and the interaction of Aly with the 3′-end processing factor Pcf11 indicates its recruitment to TREX might also be coupled with pre-mRNA 3′ end processing [14] . We suggest that TREX assembly provides a mark on mRNA to signify that nuclear RNA processing events are complete and Nxf1 deciphers this mark and exports the processed mRNA to the cytoplasm. Of considerable interest now is to establish what other nuclear processes might make use of this molecular timer as recent reports suggest that siRNA production in plants also requires the TREX complex [40] , [41] . Reagents and cell lines FLAG-Nxf1 and FLAG-Nxf1 (10RA) contain the wild-type and mutant Nxf1 cDNA, respectively, subcloned into p3XFLAG-myc-CMV-26 expression vector (Sigma) [6] . GST-Nxf1:p15 comprises the Nxf1 cDNA subcloned in pGEX6P1 (GE Healthcare) and this was cotransformed into E. coli BL21 RP strain with the p15 cDNA subcloned in pET9 (Novagen) for expression of the Nxf1:p15 heterodimer [6] . GB1-6His-Aly [6] contains ALYREF2 cDNA subcloned into pET24b containing the GB1 solubility tag. FLAG-eGFP [42] contains the EGFP gene subcloned into p3XFLAG-myc-CMV-26 expression vector (Sigma). Mutations in Nxf1 were generated by Quikchange mutagenesis following the manufacturer's instructions (Stratagene). The Nxf1 cDNA encoding aa 1–550 (Nxf1ΔUBA mutant) was amplified by PCR and cloned on an Nde I/ Xho I fragment into pET24b-GB1 [20] . The open-reading frame of Thoc5 was cloned on an Nde I/ Xho I fragment into pET24b. A cDNA fragment of the D. melanogaster Nxf1 gene corresponding to amino acids 1–112 was amplified by reverse transcriptase–PCR using RNA isolated from fly strain W 1118 using the following oligonucleotides: 5′-GAATTCCATATGCCCAAACGCGGCGGTGGCAGTA-3′ and 5′-GGCGGATCTCGAGTTAGCCAAAGCTGTTGGGCATCAGTTTGCCG-3′. The cDNA fragment was cloned on an Nde I/ Xho I fragment into pET24b-GB1 as described in Hautbergue [20] . GB1-His-tagged proteins were purified on TALON® resin following the manufacturer's instructions (Clontech). Human inducible FLP-In T-REX 293 RNAi cell lines were constructed as described previously [20] using the following target sequences: Aly no. 5 (5′-CCGATATTCAGGAACTCTTTG-3′), Thoc5 no. 1 (5′-GGCAAGGATGTGGCAATAGAA-3′), Thoc5 no. 2 (5′-TTTGTTCAGGCCACTGCGTAT-3′), Thoc2 no. 1 (5′-AAGCATGAACAGGCATCTAAT-3′), Thoc2 no. 3 (5′-TCTACAGAGATTGAAACTGGA-3′), Nxf1 no. 1 (5′-GAACACGATGATGAACGCGTT-3′), Nxf1 no. 3 (5′-GATGACATGTCTAGCATTGTT-3′). Hairpins Thoc5 no. 1 and Thoc5 no. 2, Thoc2 no. 1 and Thoc2 no. 3, Nxf1 no. 1 and Nxf1 no. 3 were chained following the manufacturer's (Invitrogen) instructions by using Bgl II and Xho I sites and Bam HI/ Bgl II compatible ends. These combinations of hairpins were further chained with Aly hairpins using the same principle to generate Aly+Thoc5 or Aly+Thoc2 targeting constructs. miRNA expression was induced with 1 μg ml −1 tetracycline (Sigma), concomitantly inducing the expression of EmGFP [20] . The Hpr1 and Nxf1 monoclonal antibodies were from Abcam and both used at 1:1,000 for western blotting. Nxf1 antibody was also used at 1:500 for immunofluorescence. The anti-Aly, anti-FLAG, anti-tubulin and anti-6His monoclonals were from Sigma and used for western blotting at 1:20,000, 1:5,000, 1:5,000 and 1:2,000, respectively. A polyclonal antibody to Thoc5 was raised against 6His-Thoc5 ( Supplementary Fig. S7 ) and used in western blotting at 1:2,000 dilution. The Thoc2 [10] and UAP56 [20] antibodies were used at dilutions of 1:1,000 and 1:2,000, respectively. FLAG-agarose and FLAG peptide were from Sigma. Sequential IPs Dishes (10×10 cm) of 293T cells were each transfected with either 18 μg of FLAG-Nxf1 or FLAG-eGFP vectors. Forty-eight hours after transfection, each dish was lysed in 1 ml of IP lysis buffer (50 mM HEPES pH 7.5, 100 mM NaCl, 1 mM EDTA, 1 mM dithiothreitol, 0.5% TX and 10% glycerol)+10 μg ml −1 RNase A). The cleared extracts were incubated with 150 μl of α-FLAG-agarose beads for 1 h. The beads were then washed with 3×5 ml of IP lysis buffer and the bound proteins were subsequently eluted in 1 ml of IP lysis buffer+FLAG peptide 100 ng μl −1 ). Fifty micro litre of polyclonal α-Thoc5 was bound to 30 μl of protein G-Sepharose. The eluate from the first IP was incubated with these α-Thoc5-beads for 1 h. The beads were then washed with 3×900 μl of IP lysis buffer. The bound proteins were finally eluted from the protein G-Sepharose with 70 μl of (0.2 M glycine pH 2.8, 1 mM EDTA), and analysed by SDS–polyacrylamide gel electrophoresis (PAGE) (10–12%) and western blot with the indicated antibodies. GST-pulldown experiments For oligo(dT) pulldown assays the indicated GST-fusion constructs were expressed and purified using glutathione sepharose according to the manufacturer's instructions (GE Healthcare). The binding reactions were performed in 0.4–1 ml of either PBS-T buffer (1×PBS, 0.1% Tween) for Nxf1 domains interactions or RB100 buffer (25 mM HEPES pH 7.5, 100 mM KOAc, 10 mM MgCl 2 , 1 mM dithiothreitol, 0.05% TX, 10% glycerol) when Thoc5 or Aly were present and for Figs 1c and 2d . Both buffers contained RNase A (10 μg ml −1 ) and subsequent washes used the same buffers containing RNase A. The pulldown in Fig. 2d also contained 0.05% bovine serum albumin as blocking agent and bound proteins were eluted from the immunoglobulin G beads using 1% SDS at room temperature. For Fig. 5b , the pulldowns were performed in PBS-T buffer-containing RNase A. The bound proteins were then washed first with PBS-T buffer, then RB100 buffer and then eluted with 50 mM Tris–HCl (pH 8.2), 40 mM GSH reduced and 100 mM KOAc. The subsequent ultraviolet-crosslinking of the eluted (GST-NTF2L:p15+6His-RBD-ψRRM-LRR) complexes or of free 6His-RBD-ψRRM-LRR with radiolabeled RNA was performed in this elution buffer and as described below. For the GST-pulldown experiments presented in Fig. 1c, 1 ml of E . coli total cell extract (6 mg ml −1 ) containing Nxf1:p15 or Nxf1ΔUBA:p15 were used and proteins detected by Coomassie staining and western blotting as indicated. For the NTF2L:p15 competitor used in the pulldown assay in Fig. 2d , GST-NTF2L:p15 was first purified on glutathione-coated beads (GE Healthcare) before on-bead cleavage with Prescission Protease. Cleaved and diluted NTF2L:p15 was desalted on G25 (GE Healthcare) in 20 mM Tris pH8.0, 25 mM NaCl before further purification on a 1-ml Mono-Q column (GE Healthcare). Resulting NTF2L:p15 was dialysed against RB100 buffer. Oligo(dT) pulldown assays For transfection-based assays, one 6-cm dish of 293T cells per condition was used and was transfected with 6 μg of the desired FLAG construct for 48 h. For assays involving endogenous proteins, one 15-cm dish per cell line or condition was used. Cells were UV-crosslinked in PBS with 300 mJ cm −2 and then lysed in the IP lysis buffer described above. The extracts were cleared by centrifugation at 16,100 g for 5 min. One (for transfection-based assays) or 2 mg (for endogeneous proteins assays) of total proteins were denatured in binding buffer (10 mM Tris–HCl pH 7.5, 0.5 M NaCl, 0.5% SDS and 0.1 mM EDTA) then incubated with 25 μl (bed volume) of oligo(dT)-cellulose beads (Sigma) for 1 h at room temperature. The beads were then washed with 3×900 μl of binding buffer. The mRNPs were finally eluted for 30 min in (10 mM Tris–HCl pH 7.5, 1 mM EDTA and 50 μg ml −1 RNase A), analysed by SDS–PAGE and western blotting with the indicated antibodies. UV-crosslinking experiments A 5′-radiolabeled 15-mer RNA (5′-CAGUCGCAUAGUGCA-3′) described previously [42] was incubated with the indicated proteins for 15 min on ice in 20 μl of RNA-binding buffer (15 mM HEPES pH 7.9, 0.2 mM EDTA, 5 mM MgCl 2 , 0.05% Tween-20, 10% glycerol and 100 mM NaCl). The reactions were then UV-irradiated for 10–15 min on ice and then analysed by SDS–PAGE. The gels were dried and the results were visualized by phosphorimaging. The UV-crosslinking experiment from Fig. 4a was done essentially as described previously [6] . Nine nanogram of 15-mer RNA was incubated for 10 min at room temperature with 50 μg of Aly alone or 5 μg of Thoc5 alone, or a combination of both Aly and Thoc5 before adding 2.5 μg of immobilized GST-Nxf1:p15. After pulldown, the beads were washed to remove unbound RNA and proteins, and eluted complexes were UV-irradiated on ice. Complexes were analysed by SDS–PAGE, stained with Coomassie blue and phosphorimaging. Fluorescence in situ hybridisation Cells grown on coverslips were fixed at room temperature for 30 min with 11.1%. paraformaldehyde in PBS. Cells were washed in PBS then incubated for 2 h at 37 °C with hybridisation solution (20% formamide, 2×sodium saline citrate, 10% dextran sulphate and 1% bovine serum albumin) containing 1 ng μl −1 Cy3-labelled oligo (dT) 50 , 0.5 μg μl −1 single-stranded DNA and 0.5 μg μl −1 tRNA and subsequently washed three times using PBS before mounting on glass slides for microscopy analysis. Immunostaining Stable 293 cell lines were fixed in paraformaldehyde and permeabilized with TX 72 h after induction of the expression of miRNAs targeting the specified genes. When indicated (+TX), the cells were treated with 0.5% of TX for 1 min on ice before fixation and immunostaining. The fluorescence intensity scans were performed on the indicated cells using the ImageJ software (NIH) with a line width of 10 and a length of 100. How to cite this article: Viphakone, N. et al . TREX exposes the RNA-binding domain of Nxf1 to enable mRNA export. Nat. Commun. 3:1006 doi: 10.1038/ncomms2005 (2012).